Local models of fractional quantum Hall states in lattices and physical implementation The fractional quantum Hall effect is one of the most striking phenomena in condensed matter physics. It is described by a simple Laughlin wavefunction and has been thoroughly studied both theoretically and experimentally. In lattice systems, however, much less is currently known, and only few models and mechanisms leading to it have been identified. Here we propose a new way of constructing lattice Hamiltonians with local interactions and fractional quantum Hall like ground states. In particular, we obtain a spin 1/2 model with a bosonic Laughlin-like ground state, displaying a variety of topological features. We also demonstrate how such a model naturally emerges out of a Fermi–Hubbard-like model at half filling, in which the kinetic energy part possesses bands with non-zero Chern number, and we show how this model can be implemented in an optical lattice setup with present or planned technologies. The fractional quantum Hall (FQH) effect [1] is one of the most fundamental phenomena in strongly correlated electronic systems and a paradigm of topological behaviour. It has been thoroughly studied and characterized in situations, where the solid surrounding the electrons has a modest effect on their properties [2] , [3] . This was possible, in part, thanks to the successful description in terms of the celebrated Laughlin wavefunctions [4] . The appearance of FQH behaviour when the lattice structure created by the solid becomes important is however not so deeply studied or understood. Nevertheless, the interest in lattice systems [5] , [6] , [7] , [8] , [9] , [10] , [11] , [12] has been sparked by the possibility of observing such behaviour with ultracold atoms in optical lattices [13] , [14] , [15] , [16] , [17] , [18] , obtaining high-temperature fractional quantum Hall states [19] , [20] , [21] , [22] , or even its applications in quantum information processing [23] . The relativistic FQH effect in graphene has also been in focus in recent years, and this effect has already been observed experimentally [24] , [25] . The standard route to the FQH effect in solids involves fractionally filled Landau levels (created by a strong, external magnetic field) and electron–electron interactions. This mechanism can be adapted to lattice systems by replacing the fractionally filled Landau level by a sufficiently flat and fractionally filled Chern band and adding near-neighbour interactions [19] , [20] , [21] , [22] , [26] , [27] (the so-called flat band models). A Chern band can be obtained by a proper choice of complex hopping amplitudes [5] and can be made flat with longer range hoppings [19] , [28] , [29] . Here we propose and investigate a different approach to obtain FQH states in lattice systems. The approach builds on conformal field theory (CFT) combined with deformations, and we use it to derive a model for spin 1/2 particles on a square lattice with some specific short-range interactions. As we will show, the ground state of the system is extremely well described by the Kalmeyer–Laughlin (KL) wavefunction [30] , [31] (the spin version of the bosonic Laughlin wavefunction with Landau level filling factor ν=1/2) and exhibits the topological behaviour expected for FQH states. In particular, we consider periodic boundary conditions and analyse the ground state (quasi) degeneracy, its response to twisting the boundary conditions, the many-body Chern number, the local indistinguishability of the ground states and the topological entanglement entropy. We also show that our model can be derived from a Fermi–Hubbard-like model, and we use this insight to propose an alternative mechanism for obtaining FQH states in lattices. Finally, we demonstrate how our model can be implemented with ultracold atoms in optical lattices. The temperatures, tunnelling amplitudes and interactions required to observe the exotic topological behaviour are the same as those required to observe the Néel antiferromagnetic order in the standard Fermi–Hubbard model, so that our predictions can be tested with present or planned technology [32] , [33] , [34] , [35] , [36] . Two perspectives on the proposed model The mechanism leading to the FQH properties can be viewed from two perspectives. The first perspective leans itself on the facts that states with interesting (topological) properties can be constructed from correlators of chiral conformal fields [11] , [37] , [38] and that nonlocal parent Hamiltonians can be derived for a quite broad class of such states [38] . We demonstrate here for the particular case of correlators from the SU (2) 1 Wess–Zumino–Witten model that the nonlocal parent Hamiltonian can, in fact, be deformed into a local Hamiltonian without crossing a phase transition, and this leads to the proposed model. The second perspective considers spin 1/2 fermions moving on a lattice with (not necessarily flat) Chern bands and strong local interactions. When the lattice filling factor is 1/2 for both spin up and spin down, a Mott state is formed, and the spin state inherits the topological character of the Chern bands. The first perspective suggests natural generalizations to other models (for example, to Moore–Read [37] -like states), and in the present paper, we propose the CFT construction combined with the idea of deforming the nonlocal parent Hamiltonian as a general strategy to construct lattice models with interesting physical properties and only local interactions. A side advantage of this approach is that the ground state of the original Hamiltonian is known (analytically or expressed as a correlator), and this is a great help to determine the physical properties of the phase in question. The local model with a KL-like ground state that we derive below demonstrates the applicability of the approach. We choose, rather arbitrarily, to define the model on a square lattice, but we note that the CFT construction allows any lattice in two dimensions (2D) to be considered. We find that the deformation of the Hamiltonian, in fact, changes the ground state very little, and we can therefore use the ground state of the original Hamiltonian as an analytical approximation to the ground state of the local Hamiltonian. This is a significant advantage compared with models in which only the Hamiltonian is known analytically. The second perspective arises because the considered model can also be derived from a Fermi–Hubbard-like model in a certain parameter regime, as we shall demonstrate. This provides additional insight and, in particular, enables us to compare our model with flat band models. The comparison shows that the properties of the Fermi–Hubbard-like model differ from those of the flat band models, which is interesting, because it opens new directions in the search for FQH states in lattices. We also use the second perspective for proposing a scheme to implement the model in ultracold atoms in optical lattices. Realizing a FQH state in optical lattices would give unique possibilities for detailed experimental investigations of the state under particularly well-controlled conditions and would, in addition, be a hallmark for quantum simulation. Model Referring back to the first of the two perspectives mentioned above, our starting point is a chiral CFT correlator which we intend to interpret as a spin wavefunction of N spins sitting at fixed positions in the 2D plane. In this construction, the chiral conformal field ( z n ) with spin j n represents the n th spin at the position (Re( z n ),Im( z n )) with internal spin state s n and spin quantum number j n . s n can take 2 j n +1 different values, and denotes the vacuum expectation value. In the following, we shall take ( z n ) to be the chiral spin 1/2 field of the SU (2) 1 Wess–Zumino–Witten model and choose s n /2=±1/2 to be the third component of the spin. In this case, (1) evaluates to [39] for N even, where δ s =1 for and δ s =0 otherwise and is the Marshall sign factor. The correlator is zero for N odd, and we shall thus take N to be even throughout. It has been found in a previous study [11] that the state (2) is closely related to the KL state and reduces exactly to it in the case of a square lattice of infinite extent. In the following, we shall refer to (2) as the CFT state in the plane. A nonlocal, exact parent Hamiltonian of has been derived in previous studies [11] , [38] by utilizing the CFT properties of the state. The Hamiltonian consists of interactions between all pairs and triples of spins in the system and is simpler than the six-body parent Hamiltonians of the exact KL state with periodic boundary conditions derived earlier [7] , [9] . The long-range interactions can be challenging to achieve experimentally. One may argue however that deforming the Hamiltonian will not dramatically change the physical properties of the ground state as long as no phase transition is crossed. With this in mind and specializing to an L x × L y square lattice with L x even, we investigate the local Hamiltonian that remains after removing all long-range interactions and making all coupling strengths position independent: Here is the spin operator of the n th spin. As indicated in Fig. 1a , the first (second) two-body term is summed over all pairs of nearest (next-nearest) neighbour spins, and the three-body term, which breaks time reversal symmetry, is summed over all triangles of neighbouring spins (for each triangle only one term is included and n , m , p label the vertices of the triangle in the counter clockwise direction as indicated with the arrow). The Hamiltonian conserves the total spin and is hence SU (2) invariant. In the following, we shall parameterize the coupling strengths as J 2 = J cos( φ 1 )cos( φ 2 ), J ′ 2 = J sin( φ 1 )cos( φ 2 ) and J 3 = J sin( φ 2 ). 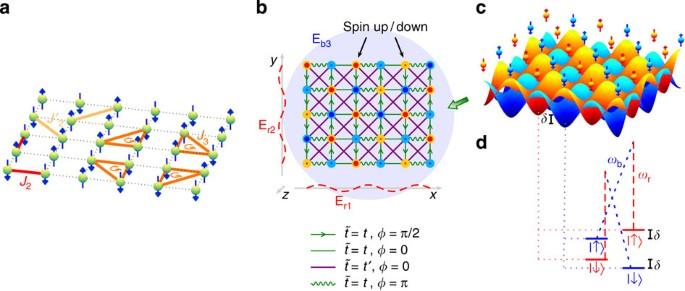Figure 1: Model and implementation. (a) The considered spin lattice Hamiltonian (3) is a sum of local two- and three-body interactions. (b) For suitable parameters, it is effectively equivalent to the Fermi–Hubbard-like Hamiltonian in equation (5), of which we here show the kinetic energy partsHkin,σ,σε{↑, ↓}. Specifically, each arrow/line/wiggle from positionntomon the lattice represents the contributiontoHkin,σwithand φ given in the figure. (c)Nfermions trapped in the optical lattice potential we propose to use for implementing the Fermi–Hubbard-like Hamiltonian. (d) We encode the spin-up and -down states in four internal hyperfine levels of the fermions. The blue/red states feel the blue/red potential in (c) and are hence trapped at the blue/red lattice sites. In this setting, we can implement the nearest-neighbour hopping terms through Raman transitions as indicated with the dashed blue and red lines in (d). For this we need the three standing wave laser fields shown in (b).Er1andEr2are directed along thex- andyaxis, respectively, and are illustrated with the red dashed lines.Eb3is directed along thezaxis and is illustrated with the blue round shadow (explicit expressions for the fields are given in Table 3). The next-nearest-neighbour hopping terms are implemented as a combination of hops induced by the fields listed above and tunnelling between nearest-neighbour sites in the blue/red lattice. Figure 1: Model and implementation. ( a ) The considered spin lattice Hamiltonian (3) is a sum of local two- and three-body interactions. ( b ) For suitable parameters, it is effectively equivalent to the Fermi–Hubbard-like Hamiltonian in equation (5), of which we here show the kinetic energy parts H kin, σ , σ ε{↑, ↓}. Specifically, each arrow/line/wiggle from position n to m on the lattice represents the contribution to H kin,σ with and φ given in the figure. ( c ) N fermions trapped in the optical lattice potential we propose to use for implementing the Fermi–Hubbard-like Hamiltonian. ( d ) We encode the spin-up and -down states in four internal hyperfine levels of the fermions. The blue/red states feel the blue/red potential in ( c ) and are hence trapped at the blue/red lattice sites. In this setting, we can implement the nearest-neighbour hopping terms through Raman transitions as indicated with the dashed blue and red lines in ( d ). For this we need the three standing wave laser fields shown in ( b ). E r1 and E r2 are directed along the x - and y axis, respectively, and are illustrated with the red dashed lines. E b3 is directed along the z axis and is illustrated with the blue round shadow (explicit expressions for the fields are given in Table 3). 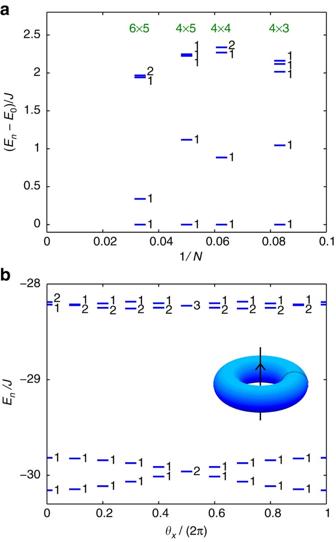Figure 3: Topological properties of the Hamiltonian. (a) Energy spectrum in the=0 subspace on the torus for different lattice sizes (in green,N=LxLy) obtained by exact diagonalization. The number to the right of each energy level is the degeneracy and only the energies of the five lowest states (n=0, 1 , 2 , 3, 4) are displayed. Note that the spectrum in the complete Hilbert space is the same except that each state is replaced by 2S+1 degenerate states, whereSis the total spin quantum number of the state. As the two lowest states haveS=0, the results suggest that there are two degenerate ground states and a gap to the first excited state in the thermodynamic limit like for theν=1/2 Laughlin state in the continuum59,60. (b) Energies of the five lowest states in the=0 subspace on the torus for twisted boundary conditions in thexdirection (θxis the twist angle) and a lattice size of 6 × 5. Twisting the boundary conditions corresponds to gradually inserting a flux line through the hole of the torus (inset), and we observe that the two ground states flow into each other under this operation.φ1=0.07 × 2π andφ2=0.03 × 2π in both panels. The next-nearest-neighbour hopping terms are implemented as a combination of hops induced by the fields listed above and tunnelling between nearest-neighbour sites in the blue/red lattice. Full size image To test how much the deformation of the Hamiltonian affects the ground state, we show the overlap between the ground states before and after the deformation as a function of φ 1 and φ 2 in Fig. 2 and as a function of lattice size in Table 1 . Even if the states are close, the overlap is expected to decrease exponentially with the total number of spins in the system due to the increase in Hilbert space dimension. This effect can be counteracted by considering the overlap per site, which is defined as the N th root of the overlap, and we also provide this measure in the table. The figure reveals a region with overlaps close to unity and shows that, for example, φ 1 =0.07 × 2π and φ 2 =0.03 × 2π (marked with the white circle) is a reasonable choice of parameters. The overlaps per site in Table 1 are around 0.999 for all the considered lattice sizes and seem not to decay with lattice size. These results are a strong indication that the deformation of the Hamiltonian does not bring the system to a different phase. 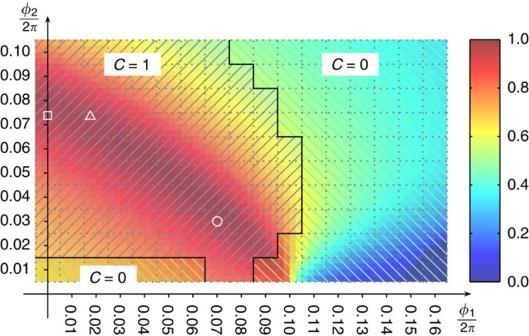In fact, we may regard equation (2) as an analytical approximation to the ground state, which is extremely helpful to see the underlying physics and to perform computations for systems that are too large for exact diagonalization. Figure 2: Phase diagram. Phase diagram of the Hamiltonian in equation (3). The background colour gives the overlap between the CFT state in equation (2) and the ground state of the Hamiltonian in equation (3) for a 4 × 5 lattice with open boundary conditions.Cis the total Chern number of the statesψ′T0andψ′T1on a 4 × 5 lattice with periodic boundary conditions, whereψ′T0(ψ′T1) is the lowest energy state in the subspace spanned by all states with the same eigenvalues ofand the translation operators in thex- andydirections as(). Within the topological phase (C=1), the two states are well separated from higher energy states in the same subspaces and flow into each other under flux insertion (like inFig. 3b). The white square, triangle and circle mark possible parameter choices considered in the text. We omitφ2=0 because the additional symmetries present for this case may cause the lowest energy states in the considered subspaces to be degenerate. Figure 2: Phase diagram. Phase diagram of the Hamiltonian in equation (3). The background colour gives the overlap between the CFT state in equation (2) and the ground state of the Hamiltonian in equation (3) for a 4 × 5 lattice with open boundary conditions. C is the total Chern number of the states ψ ′ T0 and ψ ′ T1 on a 4 × 5 lattice with periodic boundary conditions, where ψ ′ T0 ( ψ ′ T1 ) is the lowest energy state in the subspace spanned by all states with the same eigenvalues of and the translation operators in the x - and y directions as ( ). Within the topological phase ( C =1), the two states are well separated from higher energy states in the same subspaces and flow into each other under flux insertion (like in Fig. 3b ). The white square, triangle and circle mark possible parameter choices considered in the text. We omit φ 2 =0 because the additional symmetries present for this case may cause the lowest energy states in the considered subspaces to be degenerate. Full size image Table 1 Quantum numbers and overlap on the plane. Full size table The model we have looked at so far is defined in the plane and hence has open boundary conditions. To investigate the topological properties of H and the CFT state, we shall also need to consider periodic boundary conditions. On the torus, that is, for periodic boundary conditions in both directions, there are two CFT states, and , and we find analytically that these are proportional to the KL states on the torus (see Methods for explicit expressions). To ensure that the states are eigenstates of the translation operators and of the operator that rotates the lattice by 90° for L x = L y , we form the linear combinations for even-by-odd lattices and for L x = L y , respectively, where l ε{0,1}. Table 2 shows that the large overlap between the ground states of H and the CFT states also hold on the torus and provides quantum numbers of the states. Table 2 Quantum numbers and overlap on the torus. Full size table Topological properties FQH states are examples of topological states, and in the following we demonstrate that H and the CFT states exhibit topological properties that fit the properties of the ν =1/2 Laughlin state in the continuum. Characteristic features of topological states are a ground state degeneracy that depends on the topology of the surface on which the states are defined [40] , the lack of ability to distinguish the topologically degenerate states through local measurements [40] , [41] and a non-zero topological entanglement entropy [42] , [43] . For FQH states in solids another important quantity is the Hall conductivity. The Hall conductivity is closely related to the Chern number [44] , [45] , [46] , which can also be computed for spin systems. For Laughlin states the expected behaviour is a many-body Chern number of the ground state manifold on the torus that is unity and spectral flow of the ground states into each other for certain choices of the lattice size under continuous twisting of the boundary conditions [22] , [47] . We compute the spectrum on the torus through exact diagonalization of H (see, for example, the study by Läuchli [48] for a description of the numerical approach), and the results are shown in Fig. 3a . The exponential increase of the dimension of the Hilbert space with the number of spins limits the system sizes we can consider. It is seen that the two lowest energy states approach each other as the system size is increased, and extrapolating the energy difference between the third lowest and the lowest energy state to the limit N →∞ points to the existence of a gap in the thermodynamic limit. Figure 3: Topological properties of the Hamiltonian. ( a ) Energy spectrum in the =0 subspace on the torus for different lattice sizes (in green, N = L x L y ) obtained by exact diagonalization. The number to the right of each energy level is the degeneracy and only the energies of the five lowest states ( n =0, 1 , 2 , 3, 4) are displayed. Note that the spectrum in the complete Hilbert space is the same except that each state is replaced by 2 S +1 degenerate states, where S is the total spin quantum number of the state. As the two lowest states have S =0, the results suggest that there are two degenerate ground states and a gap to the first excited state in the thermodynamic limit like for the ν =1/2 Laughlin state in the continuum [59] , [60] . ( b ) Energies of the five lowest states in the =0 subspace on the torus for twisted boundary conditions in the x direction ( θ x is the twist angle) and a lattice size of 6 × 5. Twisting the boundary conditions corresponds to gradually inserting a flux line through the hole of the torus (inset), and we observe that the two ground states flow into each other under this operation. φ 1 =0.07 × 2π and φ 2 =0.03 × 2π in both panels. Full size image For finite size systems, the local indistinguishability of topologically degenerate states is not perfect, but the ability to distinguish the states decreases exponentially with the size of the system. In Fig. 4 , we plot the deviation d between the correlators of local operators computed for the two states on the torus for both the exact ground states and the CFT states. In both cases, d decreases with increasing system size, and for the CFT states the decay is clearly exponential. We also observe that d is not small unless the lattice size is at least 6 × 5. This explains why the ground state degeneracy is more pronounced for the 6 × 5 lattice in Fig. 3a than it is for smaller lattices, and the general decrease of d in Fig. 4 provides further evidence that the two lowest energies will approach each other further for larger lattices. 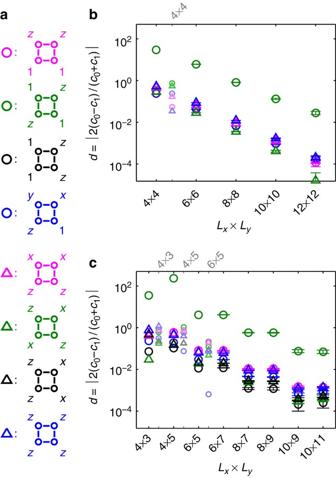Figure 4: Indistinguishability of local observables. (a) To demonstrate local indistinguishability of the states on the torus in the thermodynamic limit, we consider the set of all spin operators that act on a plaquette of four spins. Note that all plaquettes are equivalent due to the translational invariance. Using symmetries and the properties of spin operators, the correlators of all such local operators can be expressed in terms of the eight correlators depicted (the uppermost drawing, for example, represents the correlator, where the spins on the plaquette are labelledn1,n2,n3,n4in the counter clockwise direction starting from the upper right corner). For the special caseLx=Ly, the correlators displayed in black are not needed. (b) and (c), Dependence of the relative differenced=|2(c0−c1)/(c0+c1)| between the correlatorsc0≡c() andc1≡c() on the size of the lattice for even-by-even and even-by-odd lattices (we use the markers indicated in (a)). The extra set of smaller fainter symbols for 4 × 4 in (b) and 4 × 3, 4 × 5 and 6 × 5 in (c) (see the upper axes) show the same for the exact ground states of the Hamiltonian withφ1=0.07 × 2π andφ2=0.03 × 2π. The results are obtained by exact computations forLxLy≤30 and from Monte Carlo simulations forLxLy≥36. The error bars ofdare given asd±δd, where, and the variance is taken over the outcome ofindependent Monte Carlo trajectories. Figure 4: Indistinguishability of local observables. ( a ) To demonstrate local indistinguishability of the states on the torus in the thermodynamic limit, we consider the set of all spin operators that act on a plaquette of four spins. Note that all plaquettes are equivalent due to the translational invariance. Using symmetries and the properties of spin operators, the correlators of all such local operators can be expressed in terms of the eight correlators depicted (the uppermost drawing, for example, represents the correlator , where the spins on the plaquette are labelled n 1 , n 2 , n 3 , n 4 in the counter clockwise direction starting from the upper right corner). For the special case L x = L y , the correlators displayed in black are not needed. ( b ) and ( c ), Dependence of the relative difference d =|2( c 0 − c 1 )/( c 0 + c 1 )| between the correlators c 0 ≡ c ( ) and c 1 ≡ c ( ) on the size of the lattice for even-by-even and even-by-odd lattices (we use the markers indicated in ( a )). The extra set of smaller fainter symbols for 4 × 4 in ( b ) and 4 × 3, 4 × 5 and 6 × 5 in ( c ) (see the upper axes) show the same for the exact ground states of the Hamiltonian with φ 1 =0.07 × 2π and φ 2 =0.03 × 2π. The results are obtained by exact computations for L x L y ≤30 and from Monte Carlo simulations for L x L y ≥36. The error bars of d are given as d ±δ d , where , and the variance is taken over the outcome of independent Monte Carlo trajectories. Full size image In Fig. 5 , we compute the topological entanglement entropy γ using the approach proposed in a previous study [49] . For the ν =1/2 Laughlin state in the continuum, γ =ln(2)/2 (ref. 42 ), and the result we get for the CFT state is in perfect agreement with this value. For the exact ground state of H , we can again only consider rather small systems, but we observe that the results approximately follow those of the CFT state and also point to a non-zero value of γ . 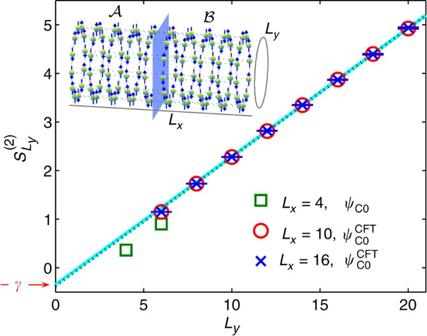Figure 5: Topological entanglement entropy. To compute the topological entanglement entropy, we map the CFT state in equation (2) to a cylinder (inset) with closed ends at ±∞ (see Methods for details). We then cut the cylinder in two halves (partand) as indicated with the blue plane, and compute the entanglement entropyas a function ofLyfor fixedLx, whereis the reduced density operator of part. We choose here to use the Renyi entropy with index 2 because it is less demanding to compute numerically than the von Neumann entropy39,56. For largeLxandLy,is independent ofLxand grows linearly withLy, and the intersection with the vertical axis is the topological entanglement entropy (−γ)42,43,49,61,62,63. The fact that the results forLx=10 andLx=16 practically coincide shows that we are already in theLx→∞ limit. The black dotted line is a linear fit to the results forLx=10 andLy≥10 and gives γ=0.374. The solid cyan line is the same fit except that γ is fixed to the value γ=ln(2)/2 ≈ 0.347 of theν=1/2 Laughlin state, and it is seen that both fits fit the data well. The results forLx=4 are computed using the lowest energy state of the Hamiltonian in equation (3) withφ1=0.07 × 2π,φ2=0.03 × 2π, and periodic boundary conditions in theydirection, and they approximately follow the results for the CFT state. The results forLx=10 andLx=16 are computed from Monte Carlo simulations of. The error bars are given as, whereand the variance is taken over the outcome ofindependent Monte Carlo trajectories. Figure 5: Topological entanglement entropy. To compute the topological entanglement entropy, we map the CFT state in equation (2) to a cylinder (inset) with closed ends at ±∞ (see Methods for details). We then cut the cylinder in two halves (part and ) as indicated with the blue plane, and compute the entanglement entropy as a function of L y for fixed L x , where is the reduced density operator of part . We choose here to use the Renyi entropy with index 2 because it is less demanding to compute numerically than the von Neumann entropy [39] , [56] . For large L x and L y , is independent of L x and grows linearly with L y , and the intersection with the vertical axis is the topological entanglement entropy (−γ) [42] , [43] , [49] , [61] , [62] , [63] . The fact that the results for L x =10 and L x =16 practically coincide shows that we are already in the L x →∞ limit. The black dotted line is a linear fit to the results for L x =10 and L y ≥10 and gives γ=0.374. The solid cyan line is the same fit except that γ is fixed to the value γ=ln(2)/2 ≈ 0.347 of the ν =1/2 Laughlin state, and it is seen that both fits fit the data well. The results for L x =4 are computed using the lowest energy state of the Hamiltonian in equation (3) with φ 1 =0.07 × 2π, φ 2 =0.03 × 2π, and periodic boundary conditions in the y direction, and they approximately follow the results for the CFT state. The results for L x =10 and L x =16 are computed from Monte Carlo simulations of . The error bars are given as , where and the variance is taken over the outcome of independent Monte Carlo trajectories. Full size image We have computed the many-body Chern number of the exact ground states on the torus for a 4 × 5 lattice as explained in Methods, and the results are depicted as a function of φ 1 and φ 2 in Fig. 2 . As the 4 × 5 lattice does not display a clear two-fold ground state degeneracy for all values of the parameters, it may happen that the two lowest energy states are not the states that resemble the CFT states. We circumvent this problem by noting that the Hamiltonian is block diagonal, which allows us to select the right states based on quantum numbers as stated in the caption. The KL states in equation (11) on the square lattice can be generalized to twisted boundary conditions by modifying the states in the same way as the ν =1/2 Laughlin states on the torus are modified when subjected to twisted boundary conditions (see equations (5.1–5.5) of the study by Read and Rezayi [50] for explicit expressions). From this we get that the many-body Chern number of the KL states on the torus for a 4 × 5 lattice is 1. Figure 3b demonstrates the flow of the ground states of H into each other when the boundary conditions are twisted, and for the KL states this property can be shown analytically. Again, our findings are thus in agreement with the properties of the ν =1/2 Laughlin state in the continuum. Finally, we note that we have done the tests above also for the parameters φ 1 =0 and (the white square in Fig. 2 ), and the results are similar. Connection to a Fermi–Hubbard-like model As mentioned in the introduction, each spin in our model may represent the spin of a fermion sitting on a site in an optical lattice. Let us consider the Fermi–Hubbard-like Hamiltonian on a square lattice, where annihilates a fermion with spin σ on lattice site n , U is a positive constant, H kin,σ is defined in Fig. 1b , and we choose the total number of fermions to equal the number of lattice sites. H kin,σ represents spin-preserving hopping of fermions between nearest and next-nearest neighbouring sites with complex hopping amplitudes, and the second term in H FH represents interactions between fermions with opposite spin sitting on the same lattice site. We note that the hopping terms give rise to a staggered flux pattern with zero total flux through the unit cell as in the Haldane model [5] . When U is much larger than the hopping strengths t , t ′, we are in the Mott insulating regime, where each site is occupied by a single fermion. In this limit, we can use the Schrieffer–Wolff transformation [51] , [52] to derive an effective Hamiltonian H eff acting in the space of states with only single occupancy on all sites in the same way as the Heisenberg model is derived from the standard Fermi–Hubbard model. Reexpressing H eff in terms of spins, we get H eff = H +constant to third order in t / U , where H is given by equation (3) with J 2 =2 t 2 / U , J ′ 2 =2 t ′ 2 / U , and J 3 =6 t 2 t ′/ U 2 . This is not by chance: the SU (2) invariance of H FH is automatically inherited to H eff and the chirality is built into the model through the complex hopping amplitudes. The choice φ 1 =0.07 × 2π and φ 2 =0.03 × 2π corresponds to t / U =0.10 and t ′/ U =0.07. Overview of simulation scheme The Fermi–Hubbard-like model can be simulated in fermions in optical lattices as follows. We encode the spin up and down states in four internal hyperfine levels as shown in Fig. 1d . By choosing the internal states appropriately and using polarized light, it is possible to construct the optical lattice in Fig. 1c , where the levels shown in blue (red) are trapped in a potential with minima located at the white (black) squares of a checkerboard. In this setup, the atoms can tunnel through the potential barrier between nearest-neighbour sites in the blue/red sublattice, which provides a contribution to the next-nearest-neighbour hopping terms in the Hamiltonian. We propose to implement the nearest-neighbour hopping terms by use of laser-assisted tunnelling [53] , [54] . This can be done with the three standing wave laser fields in Fig. 1b , which we refer to as r1, r2 and b3, respectively. As explained further below, r1 and b3 (r2 and b3) induce nearest-neighbour hops in the horizontal (vertical) direction. A hop is accompanied by a Raman transition between internal states as illustrated in Fig. 1d . The alternating signs of the hopping amplitudes originate from the spatial oscillations of the amplitudes of r1 and r2 with a period that is twice the lattice spacing, and the i ’s on the hopping amplitudes in the vertical direction appear because the amplitude of r2 is imaginary. Note that it is possible to choose the internal states in such a way that the energy difference between the blue and red spin up states is the same as the energy difference between the blue and red spin down states. r1, r2 and b3 therefore accomplish the hops for both spin up and spin down. A particularly convenient feature of the above model and implementation scheme is that only on-site interactions are needed. These occur naturally in the optical lattice, and so the Hamiltonian in equation (5) is implemented directly. Optical lattice potential The main idea behind the scheme we propose to realize the optical lattice potential in Fig. 1c is to encode the blue (red) states in internal levels that interact more strongly with right (left) circularly polarized light than with left (right) circularly polarized light and then create a checkerboard pattern of regions with highest intensity of right circularly polarized light and regions with highest intensity of left circularly polarized light. Since the blue and red sublattices are square lattices when viewed from the ( x + y ) or ( x−y ) directions, it is natural to let laser beams travel along these directions to create a standing wave pattern of intensity minima and maxima. In order to be able to control the strengths and phases of right and left circularly polarized light in the beams independently, however, the momentum vectors of the beams should have a non-zero z -component. Let us demonstrate explicitly how this can be done for fermions with one valence electron, when the ground state manifold is a 2 S 1/2 orbital, and the light fields couple the ground states off-resonantly to a 2 P 1/2 orbital as in Fig. 6a , which can be achieved with alkali atoms. We first create a standing wave pattern in the ( x + y ) direction by adding up the fields labelled 1a and 1b in Table 3 . Note that the intensity profile of the right (left) circularly polarized component of E 1a + E 1b is proportional to ( ) and that the z -polarized components of the fields are fixed by the condition that the polarization vectors of the fields must be perpendicular to the wave vectors. As seen in Fig. 6a , the presence of the z -polarized component causes the trapping lasers to induce Raman transitions between the two ground states. This undesired effect can, however, be cancelled by adding the fields 2a and 2b in Table 3 . The fields 3a, 3b, 4a and 4b do the same for the ( x − y ) direction. 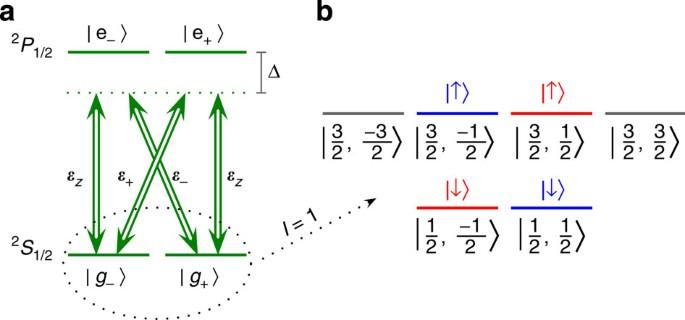Figure 6: Atomic levels and light–atom interactions. (a) Off-resonant coupling of a2S1/2ground state manifold to a2P1/2excited state manifold with polarized light. (b) Hyperfine levels of the ground state manifold when the nuclear spin isI=1. The states are labelled |F,mF›, whereFis the total angular momentum, andmFis the projection of the total angular momentum on thezaxis. The choice of blue and red spin up and down states is indicated. Figure 6: Atomic levels and light–atom interactions. ( a ) Off-resonant coupling of a 2 S 1/2 ground state manifold to a 2 P 1/2 excited state manifold with polarized light. ( b ) Hyperfine levels of the ground state manifold when the nuclear spin is I =1. The states are labelled | F , m F ›, where F is the total angular momentum, and m F is the projection of the total angular momentum on the z axis. The choice of blue and red spin up and down states is indicated. Full size image Table 3 Laser fields needed for the implementation. Full size table Eliminating the excited states with a Schrieffer–Wolff transformation, we get the trapping potentials for | g − › and | g + ›, respectively, where V 0 ∝ E 2 /(β 2 Δ), the detuning Δ, defined in Fig. 6a , and V 0 are negative (positive) for red (blue) detuning, and For − V 0 (2 β 2 + α 2 −1)>0 and − V 0 (1+2 α 2 β 2 − α 2 )>0, we thus conclude that | g − › (| g + ›) is trapped around the minima of S ( C ), which gives the desired checkerboard pattern. So far, we have considered the states at the level of fine structure. Assuming, as an example, that the nuclear spin is I =1, which is the case for 6 Li , the ground state manifold consists of six hyperfine states as depicted in Fig. 6b . The states |3/2,1/2› and |1/2,−1/2› see the potential 2 V + /3+ V − /3, and the states |3/2,−1/2› and |1/2,1/2› see the potential V + /3+2 V − /3. For suitable parameters, for example, V 0 <0 and one can therefore obtain the desired checkerboard potential by choosing the blue and red spin-up and -down states as in Fig. 6b . The states and see the potentials V + and V − , respectively, and are hence, in general, shifted away in energy, so that they can be ignored. The energy difference between the blue and red spin-up states is the same as the energy difference between the blue and red spin-down states for the above choice as desired, and this also holds when the trapping in the z -direction is taken into account. If this symmetry cannot be achieved in a given set-up, one can compensate by choosing the right and left circularly polarized components of the field b3 in Fig. 1b to have different frequencies. Note also that the energy difference between a spin sitting on a blue site and a spin sitting on a red site must be non-zero for the implementation of the hopping terms to work. If this difference is not appropriate for a given set of parameters, it can be adjusted by adding an independent standing wave laser field along the z axis with right or left circular polarization. Laser-assisted hopping The transitions induced by the fields r1, r2 and b3 in Fig. 1b can be understood by noting that the transition amplitudes are proportional to the spatial integral of the product of the Wannier functions at the two sites and the two field components that are involved in the transition. Since the Wannier functions decay rapidly, there are only transitions between nearby sites. Let us first consider the hops between neighbouring blue and red lattice sites induced by r1 and b3. The transition amplitude for hops along the y axis vanishes because the Wannier functions and b3 are even functions and r1 is an odd function with respect to reverting the x axis around the x coordinate of the sites. Hops along the x axis are allowed, and since the sign of the amplitude of r1 between two neighbouring sites is alternatingly plus and minus (see Fig. 1b ), the signs of the hopping amplitudes also alternate. r2 and b3 similarly induce hops in the y direction, but not in the x direction. For the choice of hyperfine levels considered above, it is the right (left) circularly polarized component of b3 that is involved when a fermion in the spin up (down) state hops. Therefore, one can make the hopping amplitudes for up and down spins equal by adjusting E ± appropriately, that is, by adjusting the polarization state of b3. Let us also consider transitions involving one photon from r1 and one photon from r2. In this case, the fermion cannot change its internal state due to energy conservation, and it cannot hop to a site of different colour. If the fermion remains at the same site, the transition amplitude is zero due to symmetry. If the transition involves a hop to a next-nearest-neighbour site, there is destructive interference between absorbing a photon from r1 and emitting a photon into r2 or absorbing a photon from r2 and emitting a photon into r1, and therefore no transitions occur. r1, r2 and b3 also induce transitions, where a fermion absorbs and emits a photon from the same beam without changing its internal state and either remains at the same site or hops to a next-nearest-neighbour site. The former case gives rise to the trapping in the z direction and also slightly modifies the potential in the xy plane. The modification can however be made insignificant by decreasing E r and increasing E ± without affecting the nearest-neighbour hopping amplitudes that are proportional to E r E ± . The latter case gives rise to a contribution to the next-nearest-neighbour hopping terms in the Hamiltonian. For a given choice of E ± it may happen that hops between blue lattice sites occur at a different rate than hops between red lattice sites. As mentioned above, however, one can lower the potential barriers between the sites for the sublattice with slow hops relative to the other to compensate. In the present article, we have constructed a lattice model with local interactions and a KL-like ground state and proposed a scheme for implementing it experimentally. The observation that the Fermi–Hubbard-like Hamiltonian in equation (5) captures the physics of the investigated model for provides some insight into how our model compares with previous proposals for obtaining FQH-like behaviour in lattice systems. Specifically, H FH can be seen as a sum of two free fermion models, H kin,↑ and H kin,↓ , and a local interaction term. Each of the free models has two bands of which the lowest is filled and the highest is empty. The Chern number of the filled band is plus or minus one for all non-zero t and t ′, and the band flattening, that is, the ratio of the gap between the bands to the width of either of the bands, is moderate . Our results thus show that two copies of a fermionic Chern insulator with integer band filling plus on-site interactions can give rise to a bosonic FQH state. This behaviour is different from flat band models, where a fermionic (bosonic) Chern insulator with flattened and fractionally filled bands plus interactions give rise to a fermionic (bosonic) FQH state [19] , [20] , [21] . We therefore conclude that our model provides a different mechanism to get the FQH effect in lattices. The experimental requirements to observe the desired physics in the proposed set-up are those needed to observe the Néel antiferromagnetic order in the Mott insulating regime of the standard Fermi–Hubbard model combined with the ability to perform laser-assisted hopping in a checkerboard optical lattice. Laser-assisted hopping has been demonstrated experimentally [54] , and the Fermi–Hubbard model has also been investigated experimentally. The Mott insulating regime of the Fermi–Hubbard model has been previously realized [33] , [34] , where measurements of compressibility and of the fraction of doubly occupied lattice sites were used to analyse the state. To observe the physics predicted by the effective Hamiltonian obtained by the Schrieffer–Wolff transformation, the temperature should be low compared with t 2 / U . By using a local entropy redistribution scheme, this regime has been reached for a subset of lattice bonds in a recent experiment [36] . Altogether, these results are promising for the implementation scheme proposed here. We note that the condition is needed to ensure the validity of the Schrieffer–Wolff transformation. It is possible, however, that similar physics can be observed even if H FH does not exactly reproduce the model in equation (3). This suggests that, for example, the choice t / U =1/2 and t ′/ U =1/6 (corresponding to the white triangle in Fig. 2 ), which leads to more moderate temperature requirements, may already give interesting results. The method proposed previously [38] to derive (nonlocal) parent Hamiltonians for states constructed from CFT correlators is quite general, and an interesting next step, for example, could be to apply the strategy proposed in the present paper to the Moore–Read-like state for which a parent Hamiltonian has already been derived [38] . Note added: it has been found recently in a preprint by Bauer et al. [55] that a local three-body Hamiltonian on a kagome lattice can also give rise to a state having the same topological properties as the bosonic Laughlin state at half filling. This model is, in fact, another particular case of the CFT model presented in the present paper and can be derived following the lines above using a kagome lattice rather than a square lattice. Specifically, we find that the overlaps per site between the ground states of the Hamiltonian considered previously [55] and the CFT states in equation (11) for a kagome lattice of 12 sites with periodic boundary conditions are >0.98 for both states and can be improved to values similar to those in Table 2 by adding nearest-neighbour two-body interactions. The CFT framework thus provides an analytical approximation to the ground states found numerically in the study by Bauer et al. [55] and puts their model [55] into a broader context. In addition, it is encouraging for the method presented here to observe that similar results are obtained on different lattices. Monte Carlo simulations The Monte Carlo simulations are done using the Metropolis–Hastings algorithm. To compute correlation functions we write and sample the probability distribution P ( s 1 ,…, s N )=|〈 s 1 ,…, s N |ψ›| 2 /〈ψ|ψ› as follows. We start from a random configuration s 1 ,…, s N fulfilling . In each step of the algorithm we choose a spin up and a spin down at random and flip the two spins if and only if , where is the configuration with the two spins flipped and q is a uniformly distributed random number between zero and one. Disregarding a warm-up period, the correlation function is then the average of over the trajectory. The entanglement entropy is similarly computed from the expression [39] , [56] where ( ) is shorthand notation for the spins in part ( ) of the system. The sampling is done as before, except that there are now two copies of the spins, s 1 ,…, s N and s ′ 1 ,…, s ′ N , and we therefore choose at random in each step whether we choose two spins from s 1 ,…, s N or two spins from s ′ 1 ,…, s ′ N . Wavefunction on the cylinder A cylinder with circumference L y can be mapped to the plane via the coordinate transformation z = , where ( l x , l y ) is a point on the cylinder and z is the corresponding point in the plane written as a complex number. The wavefunction for a square lattice on the cylinder is therefore easily obtained from by choosing z n = for n =1,2,…, N , where l x , n ε{−( L x −1)/2,−( L x −1)/2+1,…,( L x −1)/2} and l y , n ε{1,2,…, L y }. Wavefunctions on the torus In the spin basis, the states and take the form where k ε{0,1/2}, δ s and χ s are defined below equation (2), ω 1 and ω 2 are the periods of the torus fulfilling Im( ω 1 )=0 and Im( ω 2 / ω 1 )>0, and is the theta function. For the L x × L y square lattice, ω 1 = L x , ω 2 = iL y , and z p + L x ( q − 1 ) = p −( L x +1)/2+ i ( q −( L y +1)/2) with p ε{1,2,…, L x } and q ε{1,2,…, L y }. Note that the states in (11) are not necessarily orthogonal, but the linear combinations in equation (4) for square lattices are. Twisted boundary conditions and Chern number Let S n , m be the spin operator of the spin at position ( n , m ) on the lattice, and let . Twisted boundary conditions are then defined such that , , , and . We compute the many-body Chern number by following a previously described approach [14] , [57] . In brief, this is done by first computing ψ ′ T0 and ψ ′ T1 (defined in Fig. 2 ) as functions of θ 1 and θ 2 in the interval θ 1 , θ 2 ε[0,2π]. Let ψ ( θ 1 , θ 2 )=(| ψ ′ T0 ( θ 1 , θ 2 )›,| ψ ′ T1 ( θ 1 , θ 2 )›) and choose two sets of reference angles ( θ 1a , θ 2a ) and ( θ 1b , θ 2b ). For each zero of det( ψ † ( θ 1a , θ 2a ) ψ ( θ 1 , θ 2 ) ψ † ( θ 1 , θ 2 ) ψ ( θ 1a , θ 2a )), the increase in the phase of det( ψ † ( θ 1a , θ 2a ) ψ ( θ 1 , θ 2 ) ψ † ( θ 1 , θ 2 ) ψ ( θ 1b , θ 2b )) when going in a small circle around the zero is computed. Adding up the contributions from all the zeros and dividing by 2π gives the many-body Chern number, which is necessarily an integer. The Chern number of the bands of the free fermion model H kin, σ is computed using equation (12) of the study by Shi and Cirac [58] . How to cite this article: Nielsen, A.E.B. et al. Local models of fractional quantum Hall states in lattices and physical implementation. Nat. Commun. 4:2864 doi: 10.1038/ncomms3864 (2013).